High pressure route to generate magnetic monopole dimers in spin ice The gas of magnetic monopoles in spin ice is governed by one key parameter: the monopole chemical potential. A significant variation of this parameter could access hitherto undiscovered magnetic phenomena arising from monopole correlations, as observed in the analogous electrical Coulomb gas, like monopole dimerization, critical phase separation, or charge ordering. However, all known spin ices have values of chemical potential imposed by their structure and chemistry that place them deeply within the weakly correlated regime, where none of these interesting phenomena occur. Here we use high-pressure synthesis to create a new monopole host, Dy 2 Ge 2 O 7 , with a radically altered chemical potential that stabilizes a large fraction of monopole dimers. The system is found to be ideally described by the classic Debye–Huckel–Bjerrum theory of charge correlations. We thus show how to tune the monopole chemical potential in spin ice and how to access the diverse collective properties of magnetic monopoles. In the past two decades, remarkable technical advances have been made in pressure cell technology allowing researchers to carry out high-pressure investigations in the fields of chemistry, biochemistry, earth and planetary sciences and condensed matter physics. High pressure is used both in the laboratory and on an industrial scale to produce, for example, artificial diamonds, new superconductors and new forms of matter [1] , [2] . Pressure is also used to drive materials into new electronic states. Under high pressure, some materials become superconductors, others undergo magnetic phase transitions, and others undergo metal–insulator phase transitions [3] , [4] . In magnetic pyrochlore oxides, pressure has been shown to freeze the spin-liquid ground state of Tb 2 Ti 2 O 7 (ref. 5 ). Pressure is therefore an important weapon in a researcher's arsenal for exploring phase space. The canonical spin ices, Ho 2 Ti 2 O 7 and Dy 2 Ti 2 O 7 , with magnetic Ho or Dy ions [6] , [7] , [8] , [9] , are part of the pyrochlore family of oxides of general formula A 2 B 2 O 7 (ref. 10 ). They have face-centred cubic (fcc) lattice constants of a fcc ≈10.1 Å. These materials are not very compressible, and studies with high physical pressure have not revealed any significant modification of the spin ice properties [11] . Significantly reduced lattice constants can be obtained in principle by replacing Ti 4+ with a smaller B ion, such as Ge 4+ , but it is found that at ambient pressure the pyrochlore structure is only stable, if the ratio of the ionic radii, ρ = r A / r B , is less than 1.55 (ref. 10 ). Dy 2 Ge 2 O 7 and Ho 2 Ge 2 O 7 , with ρ ≈1.8, adopt a tetragonal structure, when synthesized under ambient pressure [12] . The range of stability of the cubic pyrochlore form can be increased using a high pressure, high temperature synthesis, which extends the regime of stability beyond ρ ≈1.8 (ref. 13 ). The cubic pyrochlore form of Dy 2 Ge 2 O 7 prepared in this way has a lattice constant of 9.9290 Å, equivalent to a canonical spin ice under enormous physical pressure [11] . The microscopic 'dipolar spin ice' Hamiltonian of Ho 2 Ti 2 O 7 and Dy 2 Ti 2 O 7 includes complex dipolar and superexchange interactions [14] , [15] . However, to a good approximation, it may be represented by a much simpler spin Hamiltonian that is equivalent to the original spin ice model [6] , [7] . In this description [9] , [14] , there are three parameters: the lattice constant a fcc , the rare earth magnetic moment μ , and an effective near-neighbour exchange parameter J eff . The equilibrium statistical mechanics then maps onto the statistical mechanics of idealized water ice, such that the low-temperature magnetic state is equivalent to the proton disordered state of water ice H 2 O (refs 6 , 7 ), and shares with it the Pauling configurational entropy [8] . The spin ice state is thus equivalent to pure H 2 O, and its excitations are equivalent to the ionic defects H 3 O + and OH − (refs 6 , 7 , 16 , 17 ). The success of this 'near-neighbour spin ice' description may be attributed to the almost perfect self-screening of the dipole–dipole interaction between rare earth moments in the effective ground state [14] . Although dipole–dipole interactions may be ignored in the spin ice ground state, in ref. 17 it was shown that inclusion of the dipole–dipole interaction in the excited states causes the 'ionic defects' of spin ice to behave as magnetic charges that interact via the magnetic Coulomb law. The description of these defects as magnetic monopoles was firmly established in ref. 16 by approximating the microscopic spin Hamiltonian Ho 2 Ti 2 O 7 and Dy 2 Ti 2 O 7 to a 'dumbbell model', where finite dipoles replace spins. The dumbbell model approximately restores dipolar corrections that are integrated out in the near-neighbour description, but still retain three parameters [16] . These are the monopole 'contact distance', (the lattice constant of the diamond lattice inhabited by the monopoles), the elementary monopole charge Q =2 μ / a (refs 16 , 17 ) and the monopole 'self-energy' ν , that replaces J eff (ref. 16 ). In ref. 18 , the self energy ν was equated with a monopole chemical potential in the grand canonical ensemble. The monopole system is a magnetic Coulomb gas of deconfined monopoles and antimonopoles with overall charge neutrality, which closely approximates a magnetic electrolyte ('magnetolyte') in the grand canonical ensemble [18] , [19] , [20] , [21] , [22] , [23] , [24] . Accordingly, experiments on the canonical spin ices reveal strong evidence of the standard field response of such a system, the Wien effect [19] , [23] , [24] , as well as of the applicability of Debye-Hückel theory in zero applied field [21] . In the magnetolyte description of spin ice, the scale of length may be set by the contact distance a and the scale of energy may be set by the Coulomb energy at contact, μ 0 Q 2 /4 πa . Different spin ices—that is, different triplets {Q, a , ν }—should have identical monopole interaction potentials if energies and lengths are scaled by the above characteristic quantities—so called 'corresponding states' behaviour. Thus, the zero-field magnetolyte properties should be fully controlled by the dimensionless temperature T *(=4 πk B T a / μ 0 Q 2 ) and the dimensionless monopole density per lattice site x ( ∝ ca 3 , where c is the concentration). These two parameters, T * and x , map out a phase space which, as mentioned above, is expected to be surprisingly rich. The x − T * phase behaviour of spin ice has not been determined in detail, but by analogy with electrolyte models [25] , [26] , [27] , we would expect a gradual transition from a weakly correlated magnetolyte at relatively large T */ x to a strongly correlated magnetolyte at small T */ x ( Fig. 1 ). However, in a given spin ice, T * and x cannot be independently varied as x is a function of T * and the chemical potential ν (Methods). Thus, any one spin ice material maps out a single trajectory in the space of x and T *, and existing spin ices are found to be firmly in the weakly correlated regime ( Fig. 1 ). In this regime, the fraction of bound monopole-antimonopole pairs is sufficiently small that it may be neglected for most purposes (the field response being an exception: see ref. 23 ). Considering, for example, Dy 2 Ti 2 O 7 , the chemical potential, ν , is found to be −4.35 K (ref. 28 ), which consists (in magnitude) of half the energy required to create a (+−) contact pair, ɛ pair / k B ≈5.7 K, plus half the energy required to unbind the pair, μ 0 Q 2 /4 πak B ≈3 K. As the dipole (+−) pair is much higher in energy than the individual (+ or −) charges, the pairing tendency is weak. In contrast, it can be seen that ν ≈3 K is the chemical potential that puts monopole–antimonopole pairs or (hetero-)dimers at the same free energy as free monopoles, and thus marks the boundary between the weakly and strongly correlated regimes ( Fig. 1 ). 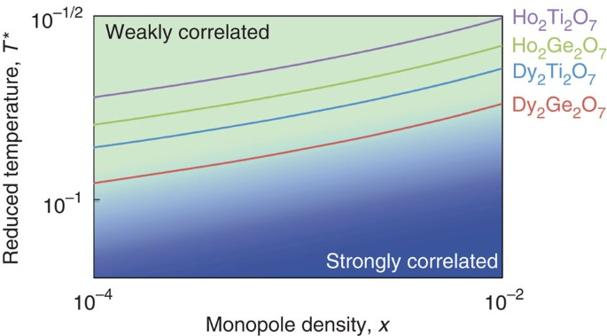Figure 1: Creating strongly correlated magnetic monopoles in spin ice. A corresponding states diagram for spin ice in terms of reduced temperatureT* and monopole density,x. A given spin ice material maps out a single trajectory but the canonical spin ices such as Dy2Ti2O7, Ho2Ti2O7lie in the weakly correlated regime (green), rather than in the strongly correlated regime (blue). By high-pressure synthesis, we have created a new spin ice Dy2Ge2O7that lies on the boundary of strong and weak correlation (red line), and hence has significant monopole dimerization at all measured temperatures (we have also created Ho2Ge2O7but this lies in the weakly correlated regime). The strongly correlated regime (lower right) has monopole correlations beyond simple pairing, potentially leading to a gas-liquid transition or charge ordering. Figure 1: Creating strongly correlated magnetic monopoles in spin ice. A corresponding states diagram for spin ice in terms of reduced temperature T * and monopole density, x . A given spin ice material maps out a single trajectory but the canonical spin ices such as Dy 2 Ti 2 O 7 , Ho 2 Ti 2 O 7 lie in the weakly correlated regime (green), rather than in the strongly correlated regime (blue). By high-pressure synthesis, we have created a new spin ice Dy 2 Ge 2 O 7 that lies on the boundary of strong and weak correlation (red line), and hence has significant monopole dimerization at all measured temperatures (we have also created Ho 2 Ge 2 O 7 but this lies in the weakly correlated regime). The strongly correlated regime (lower right) has monopole correlations beyond simple pairing, potentially leading to a gas-liquid transition or charge ordering. Full size image The only way to experimentally approach the strongly correlated regime in Figure 1 is therefore to change the chemical potential ν by changing the energy of pair creation. Fortunately, the latter depends in large part on exchange constants that vary with distance [16] . Thus a change of lattice constant from 10.1 to 9.93 Å, as achieved by substituting Ti for Ge in Dy 2 Ti 2 O 7 ( Fig. 2 ), may be sufficient to radically alter the chemical potential. We have discovered that this is indeed the case, and that Dy 2 Ge 2 O 7 , which has a much smaller lattice constant than any spin ice hitherto investigated, lies almost precisely on the boundary of the strongly and weakly correlated regimes in Figure 1 . This means that it has significant monopole dimerization at all measured temperatures. 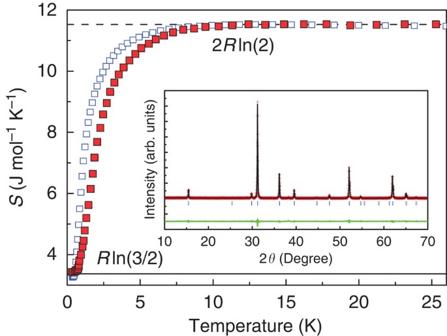Figure 2: Proof that Dy2Ge2O7(open) and Ho2Ge2O7(solid) have the characteristic Pauling zero point entropy of spin ice and water ice. The experimental molar entropy, found by integrating the magnetic specific heatCmdivided by temperatureT, when referenced to its high temperature value of 2Rln(2) per diamond lattice site, reveals a zero temperature component ofRln(3/2) equal to the Pauling value. The inset shows the Rietveld refined x-ray powder diffraction pattern of the cubic pyrochlore phase of Dy2Ge2O7with a lattice parameter of 9.9290(5) Å. Errors in the data are smaller than the symbols and represent ±1σ. Figure 2: Proof that Dy 2 Ge 2 O 7 (open) and Ho 2 Ge 2 O 7 (solid) have the characteristic Pauling zero point entropy of spin ice and water ice. The experimental molar entropy, found by integrating the magnetic specific heat C m divided by temperature T , when referenced to its high temperature value of 2 R ln(2) per diamond lattice site, reveals a zero temperature component of R ln(3/2) equal to the Pauling value. The inset shows the Rietveld refined x-ray powder diffraction pattern of the cubic pyrochlore phase of Dy 2 Ge 2 O 7 with a lattice parameter of 9.9290(5) Å. Errors in the data are smaller than the symbols and represent ±1 σ . Full size image It should be noted that the chemical potential and phase behaviour discussed here is not the same as those discussed in refs 16 , 22 in connection with a field-induced phase transition [29] . Thus the authors of ref. 16 argue that the magnetic field in that case favours ordering of positive and negative monopoles on different sublattices, leading to the phase transition, and use the terminology 'staggered chemical potential' to describe this. Experimental evidence in support of this scenario is presented in ref. 22 . However, the chemical potential we refer to is very different in that it tunes the number density of monopoles without favouring any local ordered arrangement, and is thus equivalent to the chemical potential of ions in an electrolyte (which is not true of the 'staggered chemical potential' of ref. 16 ). Pauling entropy Phase pure cubic Dy 2 Ge 2 O 7 and Ho 2 Ge 2 O 7 were prepared and characterized as described in the Methods. Here we describe our results in detail for the Dy compound only, and simply note that we have performed a similar characterization of the Ho compound, which proved to be less interesting in the present context, as it has a more typical chemical potential ( Fig. 1 ). The magnetic entropy determined by integrating the specific heat divided by temperature ( c m / T ) is shown in Figure 2 , where the Pauling residual entropy expected for spin ice [8] is extremely well reproduced. Magnetometry measurements on Dy 2 Ge 2 O 7 showed this material to have a very similar magnetic moment to Dy 2 Ti 2 O 7 . Incurring negligible error, we henceforth assume that the magnetic moment per Dy is equal in the two materials (9.87 μ B ) [15] . 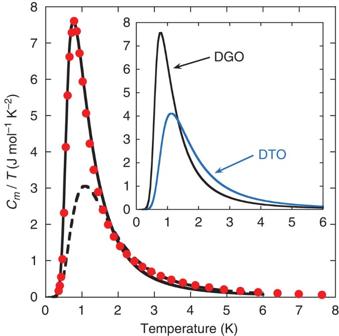Figure 3: Measured heat capacity per mole of Dy2Ge2O7at zero field compared with theoretical models. Main figure: the modified Debye-Hückel theory (Black line), with monopole chemical potentialν=3.35(5) K the only adjustable parameter, gives an excellent description of the experimental magnetic heat capacity of Dy2Ge2O7(points). Dashed black line shows the heat capacity of an ideal lattice gas with onsite exclusion with the same chemical potential. This model describes the data well at low temperatures where Coulomb interactions may be neglected, and at high temperatures where the interactions are strongly screened. Inset: the effect of varying chemical potential from −3.35 K (appropriate to Dy2Ge2O7(DGO)) to −4.35 K (appropriate to Dy2Ti2O7(DTO)). Debye-Hückel theory In Figure 3, we show the measured c m / T plotted against temperature and fitted to Debye-Hückel theory with monopole chemical potential ν =(3.35±0.05) K. The method we use has been developed to extend Debye-Hückel theory to a good approximation into the high-temperature regime; when applied to Dy 2 Ti 2 O 7 this method gives a similarly good fit to c m ( T )/ T with a chemical potential of the expected magnitude. It is based on mapping the system to a lattice gas with site exclusion. The lattice gas is considered to have a temperature-varying chemical potential equal to the sum of the true chemical potential as defined in ref. 28 and the standard Debye-Hückel Coulombic correction to the chemical potential [30] . Without the latter correction, the predicted specific heat (dotted line in Fig. 3 ) describes the experimental data well in the limit of high and low temperature, highlighting that this approach is a robust method of deriving an experimental estimate of the monopole chemical potential that is not significantly biased by the limitations of Debye-Hückel theory. In passing, we note that the origin of the approximate collapse of the experimental data and Debye-Hückel calculation onto the ideal lattice gas model at high temperature has a different origin to that at low temperature. In the latter case, the monopole gas is sufficiently dilute that interactions can be neglected, whereas in the former case, a dense and interacting monopole gas reproduces apparent ideal gas behaviour, as the result strong Coulombic screening. Figure 3: Measured heat capacity per mole of Dy 2 Ge 2 O 7 at zero field compared with theoretical models. Main figure: the modified Debye-Hückel theory (Black line), with monopole chemical potential ν =3.35(5) K the only adjustable parameter, gives an excellent description of the experimental magnetic heat capacity of Dy 2 Ge 2 O 7 (points). Dashed black line shows the heat capacity of an ideal lattice gas with onsite exclusion with the same chemical potential. This model describes the data well at low temperatures where Coulomb interactions may be neglected, and at high temperatures where the interactions are strongly screened. Inset: the effect of varying chemical potential from −3.35 K (appropriate to Dy 2 Ge 2 O 7 (DGO)) to −4.35 K (appropriate to Dy 2 Ti 2 O 7 (DTO)). Full size image As a further test for consistency, we may use our fitted value of ν to derive a value of the effective near-neighbour coupling constant, J eff , according to the relationship discussed in ref. 16 , and then compare this with a J eff estimated from the temperature of the specific heat maximum, as discussed in ref. 31 . The result is J eff =(0.62±0.1) K, (0.60±0.1) K, respectively, estimates that are equal, within experimental error. For Dy 2 Ti 2 O 7 , the corresponding value is J eff ≈1.1 K, which is roughly twice as large. The large difference is accounted for by a more negative (antiferromagnetic) exchange contribution to the spin–spin interaction in Dy 2 Ge 2 O 7 that opposes the positive (ferromagnetic) dipolar coupling, that is almost the same in the two compounds. Bjerrum pairing The measured chemical potential, −3.35 K, puts Dy 2 Ge 2 O 7 in a regime where monopole dimerization should be very significant. To confirm this, we have used the classic theory of Bjerrum [32] , who separated the contribution of closely spaced charges out of Debye-Hückel theory and regarded these as distinct chemical entities to be considered alongside the free charges. 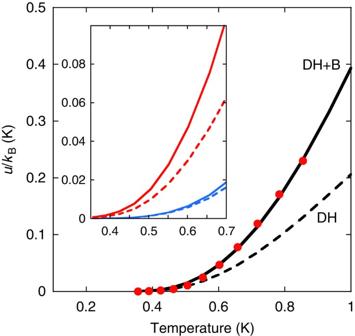Figure 4: The experimental energyu(T) of Dy2Ge2O7and the significance of the Bjerrum correction. Main figure: red circles are experimental data points. Black line is the predicted energy incorporating both free monopoles and (±) monopole dimers, using the chemical potential estimated from the data ofFigure 3. Black dashed line is the Debye-Hückel theory with a short range cutoff of two lattice spacings, which thus neglects charge dimers. However, our modified Debye-Hückel method fits the data just as well as Bjerrum's method, as it accounts for the dimers to a good approximation (Fig. 3). Inset: upper curve to lower curve are the theoretical energy for Dy2Ge2O7(with and without Bjerrum pairs) and Dy2Ti2O7(with and without Bjerrum pairs), respectively. The Bjerrum correction is much more important for Dy2Ge2O7than for Dy2Ti2O7. In Figure 4, we present the energy u ( T ) of the system found by integrating the specific heat. The result of Debye-Hückel+Bjerrum theory, as described in the Methods, is shown to give an excellent description of the low-temperature data, without the addition of any new fitting parameters. This result is not in contradiction with the fit of Figure 3 , as the modified Debye-Hückel theory described in the Methods, including the short-distance contribution of charge interactions, naturally incorporates the effect of Bjerrum pairs, to an excellent approximation. The monopoles of Dy 2 Ge 2 O 7 are found to be about 50% dimerized at all measured temperatures. Figure 4: The experimental energy u ( T ) of Dy 2 Ge 2 O 7 and the significance of the Bjerrum correction. Main figure: red circles are experimental data points. Black line is the predicted energy incorporating both free monopoles and (±) monopole dimers, using the chemical potential estimated from the data of Figure 3 . Black dashed line is the Debye-Hückel theory with a short range cutoff of two lattice spacings, which thus neglects charge dimers. However, our modified Debye-Hückel method fits the data just as well as Bjerrum's method, as it accounts for the dimers to a good approximation ( Fig. 3 ). Inset: upper curve to lower curve are the theoretical energy for Dy 2 Ge 2 O 7 (with and without Bjerrum pairs) and Dy 2 Ti 2 O 7 (with and without Bjerrum pairs), respectively. The Bjerrum correction is much more important for Dy 2 Ge 2 O 7 than for Dy 2 Ti 2 O 7 . Full size image We may put these results in the context of the corresponding states diagram (essentially the phase diagram of T * versus x ) for the restricted primitive model electrolyte, a basic model of electrolyte behaviour. In the case of a continuum electrolyte, there are three significant boundaries on this diagram marking, respectively, the onset of significant dimerization, the conductance minimum, and phase separation (see, for example, Fig. 1 in ref. 25 ). In Dy 2 Ge 2 O 7, we have reached the first of these boundaries for spin ice. To reach the other boundaries would require us to find a spin ice material with | ν | ≪ 3.3 K. However, a lattice Coulomb gas-like spin ice may show yet more complex phase behaviour in this limit, including charge-ordered phases [26] , [27] . In fact, the ultimate limit of tuning the monopole chemical potential to ν ≪ 3 K has already been identified through numerical studies on the dipolar spin ice model [14] . In monopole language, this structure consists of the ordering of 'double charges' ±2 Q to give a magnetic structure with '4 spins in/4 spins out' on alternate tetrahedra. This structure (also known as the FeF 3 structure) becomes stable at ν =2.4 K, J eff =0.2 K. In the unchartered region between ν ≈3.3 K and ν ≈2.4 K, we would expect to find a great deal of interesting physics associated with increasing monopole correlations and the gradual appearance of double charges. Our results illustrate that this region should be accessible to experiment, as we have shown how high-pressure methods afford the opportunity of dramatically altering the chemical potential of magnetic monopoles in spin ice, to the degree where new aspects of monopole physics can be revealed. Sample preparation and characterization Batches of up to 50 mg of the pyrochlore dysprosium germanate, Dy 2 Ge 2 O 7 , were made in a Walker-type, multi-anvil press. Stoichiometric amounts of Dy 2 O 3 and GeO 2 were ground thoroughly, wrapped in gold foil, compressed to 7 GPa and heated to 1,000 °C. Rietveld refinement of the X-ray powder diffraction pattern confirmed the face-centred cubic space group, (Fd-3m, No. 227) and the absence of any tetragonal pyrogermanate. The room temperature lattice parameter was determined to be 9.9290(5) Å, ( Fig. 2 (inset)). Temperature- and field-dependent magnetization measurements confirmed a rare earth magnetic moment of ∼ 10 μ B and a Curie–Weiss constant of 0.0 K. The heat capacity was measured using a thermal relaxation method between 0.34 and 25 K. The lattice contribution was subtracted from the measured specific heat to reveal the magnetic contribution. The energy u ( T ) was found by numerical integration of the measured specific heat. Heat capacity analysis To calculate the specific heat, the energy per diamond lattice site, u , was written u =| ν | x , where x is the number of monopoles per lattice site: . Here ν DH is the standard Debye-Hückel correction to the chemical potential (related to the electrochemical activity coefficient): |ν DH |/ k B T = l T /( l D + a ), where l T = μ 0 Q 2 /(8 πk B T ), is the Bjerrum length, is the Debye length, and V d is the volume per diamond lattice site (for a detailed discussion of these quantities, see ref. 23 ). Using these equations x and l D were determined self consistently, and then the specific heat was found by differentiating u . To incorporate charge dimers, we considered them as near-neighbour pairs, which is appropriate on a lattice [26] . Their chemical potential is ν d =2| ν |− μ 0 Q 2 /(4 πa ), giving the number of pairs per diamond lattice site: x B ≈2exp−| ν d |/( k B T ). The Debye-Hückel correction was modified to avoid double counting these pairs as follows: ν DH /( k B T )→ l T /( l D +2 a ). The energy was then calculated as: u =| ν d | x B +| ν | x , which was compared with the measured u ( T ). These methods have been comprehensively tested and shown to provide a robust analysis of specific heat data on spin ice materials. They were used to estimate the curves in Figures 1 , 3 and 4 . In Figure 1, the chemical potentials used are: 3.35 K (DyGe), 4.35 K (DyTi), 5.5 K (HoGe) and 5.8 K (HoTi) in an obvious notation; for the Ho materials, these are only rough estimates, owing to the difficulty of accurately isolating the electronic specific heat from the nuclear component [9] . How to cite this article: Zhou H. D. et al . High pressure route to generate magnetic monopole dimers in spin ice. Nat. Commun. 2:478 doi: 10.1038/ncomms1483 (2011).